A room temperature low-threshold ultraviolet plasmonic nanolaser Constrained by large ohmic and radiation losses, plasmonic nanolasers operated at visible regime are usually achieved either with a high threshold (10 2 –10 4 MW cm −2 ) or at cryogenic temperatures (4–120 K). Particularly, the bending-back effect of surface plasmon (SP) dispersion at high energy makes the SP lasing below 450 nm more challenging. Here we demonstrate the first strong room temperature ultraviolet (~370 nm) SP polariton laser with an extremely low threshold (~3.5 MW cm −2 ). We find that a closed-contact planar semiconductor–insulator–metal interface greatly lessens the scattering loss, and more importantly, efficiently promotes the exciton–SP energy transfer thus furnishes adequate optical gain to compensate the loss. An excitation polarization-dependent lasing action is observed and interpreted with a microscopic energy-transfer process from excitons to SPs. Our work advances the fundamental understanding of hybrid plasmonic waveguide laser and provides a solution of realizing room temperature UV nanolasers for biological applications and information technologies. Conventional laser medium has a size limit to the half of the optical wavelength in the dielectric medium. Surface plasmon (SP) provides a solution to break this diffraction limit through storing optical energy into free-electron collective oscillations [1] , [2] , [3] . SP nanolaser has recently attracted considerable interest due to its unprecedented capability of generating intense coherent light sources in the deep-subwavelength regime, offering strong light–matter interaction and many advanced applications in nanophotonics and information technology [4] , [5] . The lasing of SP, including localized surface plasmon and propagating surface plasmon polariton (SPP), has been demonstrated in metal nanosphere cavities [6] , metal-cladding nanoresonators [7] , [8] , insulator/metal nanowaveguides [9] , [10] , [11] , [12] , [13] , [14] and coupled plasmonic crystal [15] , [16] , [17] , [18] , [19] . The plasmonic cavities exhibit ultrasmall modal volume V m ~ λ 3 /10– λ 3 /1,000 ( λ is wavelength) enabling the tailoring of the strong light–matter interaction in a variety of linear (~ Q / V m ) and nonlinear (~ Q 2 / V m or Q / V m 1/2 ) optical process, where Q is the cavity quality factor. However, due to high intrinsic metal ohmic losses and radiation leakage, particularly in visible and ultraviolet regime, the Q ranges ~10–100 which is still much smaller than their dielectric counterpart [20] , [21] , [22] , [23] . As a result, the threshold of optical-pumped visible plasmonic lasing (400–700 nm) is still nearly three orders higher than II–VI/III–VI semiconductor nanostructure photonic lasing. At such an intense excitation condition, cryogenic operation is widely adopted to promote optical gain and prevent device damages [7] , [9] , [12] , which considerably limits the practical applications. Till now, it is still a big challenge to realize low-threshold room temperature SP laser. Ultraviolet laser (200–400 nm) holds important applications from high-resolution bio-imaging, laser therapy to optical storage [24] , [25] , [26] , [27] . However, as the optical wavelength approaches to the inter/intraband transition energy (for example, ~326 nm for Ag), the intrinsic ohmic loss increases dramatically thus decreases the SP-propagating length [4] , [28] . For instance, to sustain a plasmonic lasing at 400 nm along SiO 2 /Ag film, an optical gain of ~10 5 cm −1 is needed [4] . Moreover, the rapidly increased damping loss limits a high-energy asymptote in the SPP dispersion (that is, at ~360 nm for SiO 2 –Ag film), so-called bending-back effect [29] , principally discouraging the SP-lasing action above the energy limit. Hence so far, there remains an obstacle of SP lasing below 450 nm. Recent effort on ultraviolet nanolasers particularly using metal-cladded GaN stripes or nanorods has been reported; however, the deep-subwavelength mode volume is still challenging due to a small photonic–SP modal overlap or unprohibited photonic mode [30] , [31] , [32] . The hybrid plasmonic waveguide laser device, through confining electromagnetic energy into a deep-subwavelength insulator layer with propagating SPP, exhibits particular important applications in quantum information and biophotonics for straightforward propagating route, low dissipation loss and relatively high Q -factor [4] , [6] , [33] , [34] , [35] . Here we report an intense, single-mode, room temperature optically pumped ultraviolet SPP nanolaser. The SPP lasing (~370 nm) threshold is ~3.5 MW cm −2 , which is almost 1,000 times lower than that was reported in other room temperature-visible plasmonic nanolaser. We demonstrate that the outstanding performance of the plasmonic laser device is attributed to high nanowire crystalline quality and a closed-contact planar semiconductor–insulator–metal interface, which can support efficient exciton–plasmon energy transfer, large regions of high Purcell factor and low scattering loss. Moreover, we prove a dominating exciton to SP energy channel via the evidence of incidence polarization-sensitive lasing action, revealing the concept of SPP lasing in the hybrid plasmonic waveguide nanolaser devices. Structure of low-loss ultraviolet plasmoinc laser devices In such nanolaser device, three factors are critical to realize a SP lasing in UV region: high-quality cavity, well-defined contact interface, effective photonic and plasmonic modal coupling. 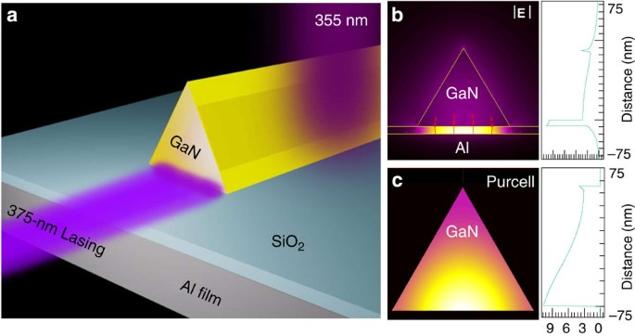Figure 1: Ultraviolet plasmonic nanolaser device. (a) Schematic of semiconductor/dielectric/plasmonic devices. GaN nanowires with a triangular cross-section is supported on Al film with 8-nm SiO2insulator separation layer. A focused quasi-continuous wave 355-nm ultraviolet laser source is used to pump the whole GaN nanowires. The GaN photoluminescence waveguides along the high-refractive nanowire, hybridize with SPP mode of Al film to produce plasmon lasing. (b) Absolute electric field (|E|) distrbutioin (left) around the plasmonic device with a wavelength ofλ=370 nm, corresponding to the lasing wavelength of GaN nanowires, calculated by a finite-element method. The electric field direction is indicated by red arrows. The |E| cross-section plot (right) confirms that the optical energy is confined into the insulating SiO2layer with a volume confinement factor of ~λ2/68. (c) Calculated local Purcell factor distribution around the GaN nanowire (left) and cross-sectional Purcell factor plots (right). Large regime inside the nanowire exhibits a Purcell factor of ~7–10. Figure 1a schematically shows the device structure consisting of a triangular GaN nanowire sitting on an aluminium (Al) film separated with a thin layer of silica (SiO 2 ). Al is adopted as the plasmonic medium due to its smaller ohmic loss in the UV regime compared with silver [24] . The gain coefficient of GaN nanowires is expected as large as ~10,000 cm −1 (refs 13 , 36 ). To reduce the interface scattering loss, the evaporation condition of Al and SiO 2 film is optimized to obtain a flat and continuous surface with a root mean square surface roughness below 0.5 nm ( Supplementary Fig. 1 ) [13] . Particularly, the GaN nanowire exhibits a triangular cross section, which constructs a fully planar semiconductor–insulator–metal interface. The edge and interface scattering loss within the planar interface is significantly suppressed, compared with a point interface in cylindrical nanowire dielectric-metal structures [9] , [13] . Moreover, the large contact area ensures a larger photonic–plasmonic modal overlap and implements an effective energy-transfer channel of exciton–plasmon coupling (see details in Discussion), to make full use of the optical gain from semiconductor. Figure 1: Ultraviolet plasmonic nanolaser device. ( a ) Schematic of semiconductor/dielectric/plasmonic devices. GaN nanowires with a triangular cross-section is supported on Al film with 8-nm SiO 2 insulator separation layer. A focused quasi-continuous wave 355-nm ultraviolet laser source is used to pump the whole GaN nanowires. The GaN photoluminescence waveguides along the high-refractive nanowire, hybridize with SPP mode of Al film to produce plasmon lasing. ( b ) Absolute electric field (| E |) distrbutioin (left) around the plasmonic device with a wavelength of λ =370 nm, corresponding to the lasing wavelength of GaN nanowires, calculated by a finite-element method. The electric field direction is indicated by red arrows. The | E | cross-section plot (right) confirms that the optical energy is confined into the insulating SiO 2 layer with a volume confinement factor of ~ λ 2 /68. ( c ) Calculated local Purcell factor distribution around the GaN nanowire (left) and cross-sectional Purcell factor plots (right). Large regime inside the nanowire exhibits a Purcell factor of ~7–10. Full size image Figure 1b shows the simulated cross-sectional electric field distribution of the GaN–SiO 2 –Al structure ( λ ~370 nm, Methods). The GaN nanowire-edge length a is ~100 nm. The electromagnetic energy is concentrated in the thin 8-nm insulator gap region, exhibiting a deep-subwavelength modal volume of ~ λ 2 /68 (Methods). On the other hand, the confinement factor in the GaN nanowire is ~3.42, indicating that a high percentage of the bulk material gain supplied by the GaN nanowire is harnessed in this hybrid configuration. The local Purcell factor distribution inside the GaN nanowires is displayed in Fig. 1c , suggesting that most of the GaN nanowire regime exhibits a pronounced Purcell factor of ~7–10, supporting the effective coupling between the semiconductor waveguide and the SPP mode. Lasing characterization of plasmonic device The plasmonic laser device ( Fig. 2a ) is optically pumped by a 355-nm nanosecond-pulsed laser (Methods). The incident polarization is made to be circular to eliminate the emission polarization response to excitation, and the emission light along and perpendicular to the nanowire long axis ( c ) is collected individually ( Fig. 2b ). Below the lasing threshold ( I ex ~0.5 MW cm −2 ), pronounced Fabry–Pérot oscillations (arrows, Fig. 2c ) can be resolved over a broad band-edge emission band of GaN nanowires (370 nm, room temperature), suggesting the observation of the longitudinal cavity modes resonated between two nanowire-end facets. The emission intensity along the nanowire axis (red curve, Fig. 2c ) is stronger than the perpendicular component (blue curve, Fig. 2c ), manifesting the dominate waveguiding of SPP in the cavity. A high group refractive index n g of 7.61 is extracted ( Fig. 2c , inset), which agrees well with our calculation ( n g ~8.96, Methods). The group index can be further increased with the pumping fluence and decreasing of the nanowire diameter due to a higher carrier density, stronger coupling and larger loss [9] , [10] . 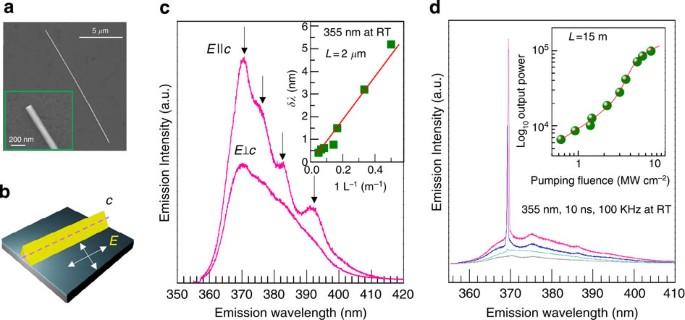Figure 2: Room temperature ultraviolet plasmonic lasing characterization. (a) Scanning electron microscopy (SEM) image of a GaN nanowire sitting on SiO2/Al film. Inset: magnified scanning electron microscopy image of one end of the GaN nanowire. The nanowire length and diameter is 15 μm and 100 nm, respectively. (b) Schematic of optical measurement and polarization detection setup.cis defined as the orientation of nanowire. The incidence excitation laser is circular polarized and the focused laser beam can cover the whole nanowire. The emission scattered out from two ends is collected and the polarization property along and perpendicular to nanowire axiscis analysed. (c) Spontaneous emission of as-fabricated plasmonic device below lasing threshold at room temperature under a power fluence of 0.5 MW cm−2. Arrows highlight the Fabry–Pérot peaks. The nanowire length is 2 μm. Inset: cavity mode spacingδλvariation with nanowire lengthL(green dots).δλversus 1/Lcan be well fitted with a linear function (red curve), suggesting a high group indexng(ng=λ2/2L) of 7.61 due to the high gain requirement of the plasmonic laser device. (d) Power-dependent emission spectra of the plasmonic devices. One sharp peak with a maximum full width at half maximum (FWHM) ~0.8 nm appears above the spontaneous emission background. The nanowire length is 15 μm. Inset: integrated emission versus pumping intensity. TheS-shaped plot suggests the evolution from a spontaneous emission, amplified spontaneous emission to lasing process. Figure 2: Room temperature ultraviolet plasmonic lasing characterization. ( a ) Scanning electron microscopy (SEM) image of a GaN nanowire sitting on SiO 2 /Al film. Inset: magnified scanning electron microscopy image of one end of the GaN nanowire. The nanowire length and diameter is 15 μm and 100 nm, respectively. ( b ) Schematic of optical measurement and polarization detection setup. c is defined as the orientation of nanowire. The incidence excitation laser is circular polarized and the focused laser beam can cover the whole nanowire. The emission scattered out from two ends is collected and the polarization property along and perpendicular to nanowire axis c is analysed. ( c ) Spontaneous emission of as-fabricated plasmonic device below lasing threshold at room temperature under a power fluence of 0.5 MW cm −2 . Arrows highlight the Fabry–Pérot peaks. The nanowire length is 2 μm. Inset: cavity mode spacing δλ variation with nanowire length L (green dots). δλ versus 1/ L can be well fitted with a linear function (red curve), suggesting a high group index n g ( n g = λ 2 /2 L ) of 7.61 due to the high gain requirement of the plasmonic laser device. ( d ) Power-dependent emission spectra of the plasmonic devices. One sharp peak with a maximum full width at half maximum (FWHM) ~0.8 nm appears above the spontaneous emission background. The nanowire length is 15 μm. Inset: integrated emission versus pumping intensity. The S -shaped plot suggests the evolution from a spontaneous emission, amplified spontaneous emission to lasing process. Full size image With I ex =2.5–4.0 MW cm −2 , the output power shows a super-linear increase, with an appearance of a sharp peak (full width at half maximum (FWHM) ~0.8 nm) over the spontaneous emission background, suggesting the occurrence of amplified spontaneous emission ( Fig. 2d ). As I ex is further increased beyond 4 MW cm −2 , the spectrum is concentrated and dominant with the sharp peak (full lasing action). The integrated emission intensity including the spontaneous background I out on a log–log scale suggests a threshold of 3.5 MW cm 2 ( Fig. 2b , inset). The lasing threshold value is in good agreement with a theoretical prediction based on the loss-compensation model in hybrid plasmonic waveguide laser [37] . Moreover, the lasing threshold is three orders of magnitude lower than that of the other room temperature plasmonic nanolaser device (~GW cm −2 ) [12] . Numerical analysis of plasmonic and photonic mode How to validate the SP lasing is an important issue [18] , [19] , [38] . In this work, mode simulation, emission polarization properties and time-resolved spectroscopy are conducted to prove the observation of plasmonic lasing. Calculations on the GaN nanowire-edge length ( a ) dependence of the effective index and field distribution for the hybrid plasmonic and photonic modes are performed. The effective index n eff used to quantify the phase velocity in the direction along nanowire axis is proportional to the real part of the eigenvalue β , that is, n eff = Re { β }/ k 0 , where k 0 is the incident wave vector. In GaN–SiO 2 configuration (photonic device, Fig. 3a ), photonic modes such as HE11-like, EH11-like, TE01-like and TM01-like modes are supported if a >~220 nm ( Fig. 3c ). The electric field distribution can be seen in Supplementary Fig. 2a (ref. 39 ). If when a <~130 nm, all the four photonic modes are prohibited, as indicated by the vertical dashed line in Fig. 3c . 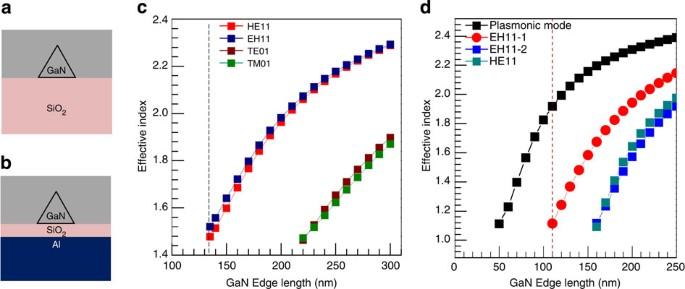Figure 3: Modes in photonic and plasmonic devices. (a,b) Simulation configuration of photonic (a) and plasmonic devices (b). Photonic device: the GaN nanowire is sitting on a SiO2substrate with infinite thickness; plasmonic device: the GaN nanowire is sitting on Al substrate with a thin SiO2(8 nm) spacer layer. (c) The effective refractive index of HE11-like (red), EH11-like (blue), TE01-like (wine) and TM01-like (oliver) mode versus the GaN nanowire-edge lengtha. The cutoff sizes of HE11-like and EH11-like mode are arounda=135 nm (dashed line). (d) The effective indexes of hybrid plasmon mode (black), photonic EH11-1-like (red), EH11-2-like (green), HE11-like (blue) modes versus the GaN nanowire-edge length in plasmonic device. The cutoff size of EH11-1-like mode is arounda=110 nm (dashed line). Figure 3: Modes in photonic and plasmonic devices. ( a , b ) Simulation configuration of photonic ( a ) and plasmonic devices ( b ). Photonic device: the GaN nanowire is sitting on a SiO 2 substrate with infinite thickness; plasmonic device: the GaN nanowire is sitting on Al substrate with a thin SiO 2 (8 nm) spacer layer. ( c ) The effective refractive index of HE11-like (red), EH11-like (blue), TE01-like (wine) and TM01-like (oliver) mode versus the GaN nanowire-edge length a . The cutoff sizes of HE11-like and EH11-like mode are around a =135 nm (dashed line). ( d ) The effective indexes of hybrid plasmon mode (black), photonic EH11-1-like (red), EH11-2-like (green), HE11-like (blue) modes versus the GaN nanowire-edge length in plasmonic device. The cutoff size of EH11-1-like mode is around a =110 nm (dashed line). Full size image In GaN–SiO 2 –Al configuration (plasmonic device, Fig. 3b ), the typical hybrid mode distributions indicate that not only the hybrid plasmonic mode but also the hybrid photonic modes can be supported (see Supplementary Fig. 2b ). However, the hybrid photonic modes, supported in the GaN–SiO 2 –Al configuration due to a large permittivity mismatch, are cutoff as a <~110 nm ( Fig. 3d ). Only one hybrid plasmonic mode exists if a is between 50 nm and ~110 nm, which suggests that the lasing action observed in Fig. 2d is due to the hybrid plasmonic mode. We notice in Fig. 3c that no photonic mode can be supported in GaN nanowire when a <~130 nm; however, it is still possible to support hybrid photonic modes EH11-1 when the nanowire is sitting on SiO 2 –Al structure ( Fig. 3d ). As a result, it is more precise to determine the cutoff size for photonic mode in the semiconductor–insulator–metal configuration instead of in the semiconductor-SiO 2 configuration as done previously [9] . Emission polarization of plasmonic and photonic lasing The longitudinal plasmonic and photonic modes exhibit distinct polarization behaviour [9] , [33] . 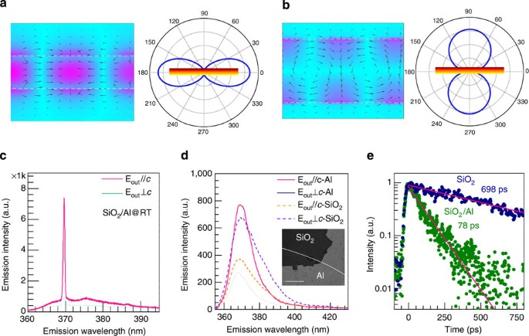Figure 4: Plasmonic lasing polarization and Purcell effect. (a,b) Hybrid plasmonic mode polarization distribution along the thin GaN nanowire (150 nm) sitting on SiO2/Al film (a), and photonic waveguide-mode polarization distribution along thick GaN nanowires (200 nm) on SiO2substrate (b). Left panels: near-field electric field and oscillation direction. Black arrows indicate the electric field direction. Dashed line indicates the nanowire edge. Right panels: far-field emission intensity as a function of polarization angle. The polarization angle is defined as the angle between electric field direction and nanowire axisc. (c) Plasmonic lasing intensity along two polarization directions. (d) Polarization-dependent spontaneous emission spectra of the same GaN nanowire sitting on SiO2/Al (solid curves) and SiO2(dashed curves) substrate along the two polarization directions. Inset: scanning electron microscopy (SEM) image of the GaN nanowire. The scalar bar is 4 μm. (e) Time-resolved two-photon-pumped emission of the GaN nanowire (d) sitting on SiO2/Al (green dots) and SiO2(blue dots). The decay curves can be well fitted by a single-exponential function with a lifetime of 78 and 698 ps for plasmonic and photonic device, respectively. Figure 4a,b presents the simulated near-field (left) and far-field (right) polarization distributions ( E -field) of the emission scattered out from the nanowire tips. In the plasmonic device (GaN–SiO 2 –Al), the electric field normal to the metal surface exhibits the strongest coupling to SPP, thus the emission is highly polarized along the nanowire axis ( Fig. 4a ). However, in photonic device (GaN–SiO 2 ), the transverse electric modes waveguide and oscillate inside the GaN nanowires, leading to a stronger emission with the polarization perpendicular to the nanowire axis ( Fig. 4b ). Experimentally, as shown by Fig. 4c , the plasmonic lasing is significantly polarized along the nanowire; while in photonic lasing mode the perpendicular component is stronger than the parallel component ( Supplementary Fig. 3 ). The polarization of plasmonic lasing, influenced by incidence polarization (discussion later) and collection angle and so on, is ~50% for E out // c which is comparable with previous works [13] , [14] . The polarization dependence of the spontaneous emission below the threshold is also observed, taken along the GaN nanowire across the Al boundary ( Fig. 4d ). The nanowire on top of SiO 2 –Al exhibits a dominating E out // c emission, while the nanowire directly sitting on SiO 2 substrate shows a dominating E out ⊥ c emission, suggesting that it is not the dielectric distinction or exciton transition but the plasmonic cavity determining the polarization [40] . To conclude, the dominating E out // c emission in plasmonic mode, supported by the cutoff size prediction discussed previously, unambiguously confirm the achievement of plasmonic lasing. Figure 4: Plasmonic lasing polarization and Purcell effect. ( a , b ) Hybrid plasmonic mode polarization distribution along the thin GaN nanowire (150 nm) sitting on SiO 2 /Al film ( a ), and photonic waveguide-mode polarization distribution along thick GaN nanowires (200 nm) on SiO 2 substrate ( b ). Left panels: near-field electric field and oscillation direction. Black arrows indicate the electric field direction. Dashed line indicates the nanowire edge. Right panels: far-field emission intensity as a function of polarization angle. The polarization angle is defined as the angle between electric field direction and nanowire axis c . ( c ) Plasmonic lasing intensity along two polarization directions. ( d ) Polarization-dependent spontaneous emission spectra of the same GaN nanowire sitting on SiO 2 /Al (solid curves) and SiO 2 (dashed curves) substrate along the two polarization directions. Inset: scanning electron microscopy (SEM) image of the GaN nanowire. The scalar bar is 4 μm. ( e ) Time-resolved two-photon-pumped emission of the GaN nanowire ( d ) sitting on SiO 2 /Al (green dots) and SiO 2 (blue dots). The decay curves can be well fitted by a single-exponential function with a lifetime of 78 and 698 ps for plasmonic and photonic device, respectively. Full size image The spontaneous emission decay rate of GaN nanowire is significantly enhanced in the plasmonic device due to Purcell effect [41] , [42] , [43] . As shown in Fig. 4e , the GaN emission lifetime, measured by a two-photon excitation (Methods), decreases from 698 (photonic device) to 78 ps (plasmonic device). The Purcell factor of ~8.9 corresponds to a mode that is a hundred times smaller than the diffraction limit, which agrees with our analytical calculations ( Fig. 1b ) and local Purcell factor distribution ( Fig. 1c ). Incidence polarization-sensitive plasmonic lasing We find that the SPP-lasing modes are sensitive to incident polarization. In the previous reports on plasmonic nanolasers, the incident polarization has not been considered [9] , [12] , [13] . Instead of using a circularly polarized laser, we use linearly polarized laser to pump the same nanowire, and to detect the lasing emission from the tip in two polarizations ( Fig. 5a ). When the incident polarization is along the nanowire ( E in // c ), the plasmonic lasing exhibits a single-mode operation centred at 369 nm, with a higher intensity along the nanowire axis ( Fig. 5b ). If the incident polarization is rotated by 90° ( E in ⊥ c ), multimode emission appears with the strongest mode red shifted to 372 nm ( Fig. 5c ), nevertheless, the polarization is still dominated by E out // c emission. However, the lasing intensity and the polarizing ratio is larger when the incident polarization is along the nanowire, indicating a more effective hybridization or a stronger coupling between the semiconductor waveguide and the SPPs. The larger modal overlap results in a better cavity quality and therefore single-mode lasing is obtained. 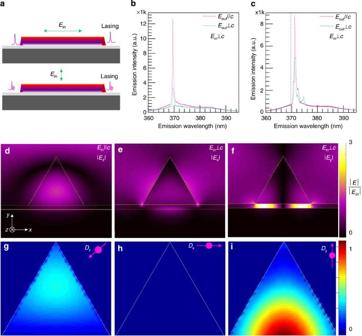Figure 5: Incident polarization selected plasmonic lasing modes. (a) Schematic of plasmonic lasing selected by incidence polarization. Linear polarization, along (upper panel) and perpendicular to (bottom panel) the nanowire axiscis used to excite the plasmonic device. Single-mode (upper panel) and multimode (bottom panel) plasmonic lasing can be obtained, respectively. (b,c) Experimental spectra when the excitation polarization is along (b) and perpendicular to (c) nanowire axisc. The red and green curves show the emission spectra along and perpendicular to the nanowire axisc, respectively. (d,f) The total incident electric field in hybrid plasmonic devices as the incident polarization is along the nanowire axisc(|Ez|, (d) and perpendicular to nanowire axisc(e) |Ex|; (f) |Ey|). (g–i) The dipole-field coupling efficiency distribution of GaN exciton dipole fields into hybrid plasmonic modes along the GaN–SiO2–Al interface. The exciton dipoles are polarized along z,x,ydirection (|Ez|,g; |Ex|,h; |Ey|,i). Figure 5: Incident polarization selected plasmonic lasing modes. ( a ) Schematic of plasmonic lasing selected by incidence polarization. Linear polarization, along (upper panel) and perpendicular to (bottom panel) the nanowire axis c is used to excite the plasmonic device. Single-mode (upper panel) and multimode (bottom panel) plasmonic lasing can be obtained, respectively. ( b , c ) Experimental spectra when the excitation polarization is along ( b ) and perpendicular to ( c ) nanowire axis c . The red and green curves show the emission spectra along and perpendicular to the nanowire axis c , respectively. ( d , f ) The total incident electric field in hybrid plasmonic devices as the incident polarization is along the nanowire axis c (| E z |, ( d ) and perpendicular to nanowire axis c ( e ) | E x |; ( f ) | E y |). ( g – i ) The dipole-field coupling efficiency distribution of GaN exciton dipole fields into hybrid plasmonic modes along the GaN–SiO 2 –Al interface. The exciton dipoles are polarized along z, x , y direction (| E z |, g ; | E x |, h ; | E y |, i ). Full size image The polarization-sensitive lasing behaviour can be well understood by combining the passive hybrid plasmonic waveguide approach with a microscopic active photon–exciton–SPP interaction model. Based on the quantum theory of plasmonic lasing [4] , [18] , [44] , the tremendous SPP transition energy to achieve population inversion in metal system is furnished by gain media via nonradiative energy transfer from excitons to SPP. Therefore, the population and coupling efficiency of exciton to the SPP mode are important to plasmonic lasing performance ( Q -factor and threshold and so on). The total electric field distribution excited by the incident pump at 355 nm, which determines the population and distribution of launched excitons, is calculated to evaluate the population and coupling efficiency. Figure 5d shows the z -component when the incident polarization is along the c axis, in which both the x - and y -components are zero. Figure 5e,f display the E x (5e) and E y (5f) components of the total excitation electric field when the incident polarization is perpendicular to c axis (355 nm), in which the z -component is zero. The dipoles in the GaN nanowire embodying the gain are assumed to be polarized parallel to the total electric field. Figure 5g–i shows the local dipole-field coupling efficiency [45] inside the GaN nanowire into hybrid plasmonic mode as a function of the position of the dipole for each polarization. Only the y - and z -polarized dipoles can couple to the hybrid plasmonic modes therefore will drive plasmonic lasing. The effective gain harvested by the hybrid plasmonic mode is then determined by multiplying the dipole population, which is proportional to the total excitation electric field intensity | E | 2 in the nanowire gain region, and the local dipole-field coupling efficiency. By integrating the effective gain inside the GaN nanowire, the total effective gain for E in // c is estimated to be ~1.87 times over that for E in ⊥ c (details in Supplementary Fig. 4 and Supplementary Discussion ), which agrees well with the corresponding ratio of measured peak emission intensity in Fig. 5b,c (about 1.46). In other words, the relatively larger effective gain harvested leads to a stronger lasing intensity when the pump polarization is along nanowire axis. Although there are experimental observations of lasing based on the hybrid plasmon waveguide devices, the claim of the SP lasing is still very controversial [38] , [46] . A fundamentally important issue, that is, whether the lasing nature is an amplification of stimulated SP emission or only a plasmon-assisted photonic lasing, has to be clarified. SPP lasing is accomplished by efficient energy transfer from exciton to SPP. However, in plasmon-assisted photonic lasing an inverse energy-transfer process is dominated, which is usually manifested as enhanced luminescence and more rapid radiative decay channels due to strong localized electromagnetic field. Our experiments of excitation-polarization-sensitive lasing behaviours suggest that the energy is transferred from exciton to SPP in hybrid plasmonic devices. To achieve plasmonic lasing, the modal loss α m must be overcompensated by the modal gain g m , such as g m > α m (refs 47 , 48 ). The loss in a plasmonic cavity α m is mainly contributed by four parts: intrinsic ohmic damping ( α e-scat , α e-h ) and extrinsic radiation ( γ rad ) and scattering losses ( γ scat ). α e-scat and α e-h is the absorption coefficient of individual free-electron scattering (with electrons, lattice ions, impurities and so on) and the inter/intraband transition for excitation of electron–hole pairs, respectively ( Fig. 6a ) [28] ; γ rad and γ scat is the radiation and scattering loss in the plasmonic cavities, respectively ( Fig. 6b ) [9] , [13] . The intrinsic ohmic loss is mainly determined by metal itself, while the extrinsic loss can be effectively reduced via clever design of the plasmonic cavities (symmetry, roughness and facet reflectance and so on). In principle, γ rad occurs primarily at the nanowire end ( Fig. 6b, I ) which can be evaluated as −2/ L × ln R , where R is the facet reflectance of SPP mode. To reduce the γ rad , long nanowire ( L =15 μm) is adopted. On the contrary, the total intrinsic ohmic loss is much larger than γ rad by nearly one order of magnitude (Methods). To further improve the Q values, smart design of high-reflective plasmonic cavity is demanded, such as using distributed Brag reflector structure. Secondly, γ scat arises via scattering of propagating SPP to localized SP or out of plasmonic cavity ( Fig. 6b. II ), which occurs mainly at rough semiconductor–insulator–metal interface [47] . In our work, the root mean square surface roughness of SiO 2 –Al and Al film is optimized down to sub-nanometers (0.454 and 0.359 nm, respectively) to minimize γ scat . Furthermore, the construction of a planar interface using triangular nanowires relatively decreases the edge-scattering ratio, which even holds a stronger confinement of electromagnetic wave inside the cavity ( Fig. 6b, III ). 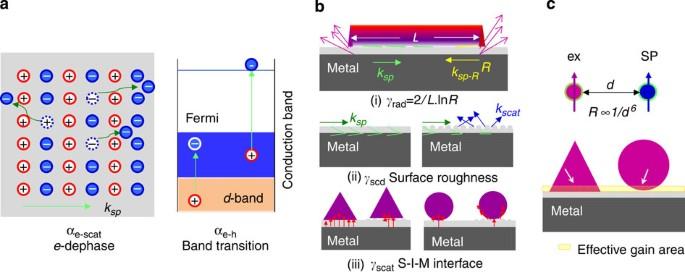Figure 6: Loss and gain in hybrid plasmonic laser device. (a) Schematic of two surface plasmon intrinsic damping (ohmic loss) channels: nonradiative dephasing of individual electron via scattering with electrons, phonons, lattice ions and impurities at low energy and so on, excitation of electron–hole pair via intra- and interband transition at high energy. (b) Schematic of extrinsic surface plasmon damping via radiative emission at cavity facet (γrad, I), scattering at rough metal surface (γscat, II) and scattering at semiconductor–insulator–metal interface (III). Higher confinement and lower scattering loss is shown for a planar semiconductor–insulator–metal interface. (c) Exciton–surface plasmon energy transfer based on a dipole–dipole interaction model (upper panel). The energy-transfer rate is proportional to the sixth power of the distance between them. Bottom panel: the effective gain area (yellow area), in two types of semiconductor–insulator–metal interface. The planar interface exhibits a larger effective area to supply optical gain to compensate the loss in metal. Figure 6: Loss and gain in hybrid plasmonic laser device. ( a ) Schematic of two surface plasmon intrinsic damping (ohmic loss) channels: nonradiative dephasing of individual electron via scattering with electrons, phonons, lattice ions and impurities at low energy and so on, excitation of electron–hole pair via intra- and interband transition at high energy. ( b ) Schematic of extrinsic surface plasmon damping via radiative emission at cavity facet ( γ rad , I), scattering at rough metal surface ( γ scat , II) and scattering at semiconductor–insulator–metal interface (III). Higher confinement and lower scattering loss is shown for a planar semiconductor–insulator–metal interface. ( c ) Exciton–surface plasmon energy transfer based on a dipole–dipole interaction model (upper panel). The energy-transfer rate is proportional to the sixth power of the distance between them. Bottom panel: the effective gain area (yellow area), in two types of semiconductor–insulator–metal interface. The planar interface exhibits a larger effective area to supply optical gain to compensate the loss in metal. Full size image Another important issue is how to harness optical gain from active media thoroughly. The plasmonic lasing process can be facilitated by three steps: an exciton in gain media is launched by the incident photons; then the excitons recombine nonradiatively and the energy is transferred to metal system via excitation of a SP; the SP stimulates the excitons in gain media to create more SPs. During the second and third steps, a high efficiency of nonradiative energy transfer between exciton and SP is critical to achieving population inversion of SP. The SP population variation can be expressed as where N ex is the exciton population, R ex−SP is the exciton–SP nonradiative energy transition rate, z is the SP propagating distance, and c is the speed of light in free space. From the equation (1), the SP mode gain is proportional to R ex−SP , which decays rapidly with the exciton–SP distance. Based on a dipole–dipole interaction model [49] , A is a constant for a given system, d is the distance between SP and exciton. As d >10 nm, the exciton–SP energy-transfer efficiency is too low to provide sufficient gain to overcompensate the SP propagating loss [50] . However as d< 5 nm, the opening of other nonradiative channels, such as electron transfer, lower the gain of active media. The speculated optimal thickness for plasmonic amplification is of the range 5~10 nm, for example, the SiO 2 insulator thickness of 8 nm deposited in this work. Furthermore, for a fixed insulator layer thickness, we believe that the effective gain compensation area of a planar interface is larger than cylindrical interface (shown in Fig. 6c ). Therefore, we believe that the low-threshold and high- Q plasmonic lasing with such a short-wavelength output mode is mainly attributed to the close-contact planar interface. Metal-insulator film deposition and characterization To reduce the radiation loss and ensure a good contact between GaN nanowire and planar plasmonic cavity, SiO 2 on Al film with small roughness is prepared. The Al film with a thickness of 100 nm was deposited onto a 300-nm SiO 2 /Si substrate by an electron-beam evaporator. The film root mean square surface roughness is ~0.359 nm measured by atomic force microscopy. The Al film is well protected in vacuum and then an insulator SiO 2 layer is deposited on to the Al film by magnetron sputtering. The total root mean square surface roughness of SiO 2 –Al film was measured to be ~0.454 nm. The SiO 2 thickness is designed to be 8 nm to form a continuous film. Nanowire synthesis and characterization The GaN nanowire was grown by metal-organic chemical vapour deposition on sapphire substrates using trimethylgallium and ammonia as Ga and N precursors, respectively, and hydrogen as a carrier gas (ref. 21 ). The previous transmission electron microscopy and scanning electron microscopy studies show that the nanowire has triangular cross-section and smooth surface. The nanowire-edge length is 100–300 nm. The smooth surface is advantage for good contact between GaN with SiO 2 –Al film. The as-grown GaN nanowires were ultrasonically removed from substrate, dispersed into isopropyl alcohol and deposited onto preprepared SiO 2 –Al films substrate. Optical characterizations The plasmonic lasing measurement was conducted using a Horiba-JY T64000 spectrometer. A quasi-continuous wave laser (pulsed width: 10 ns, repetition rate: 100 KHz) with a wavelength of 355 nm is focused by an objective ( × 40, numerical aperture: 0.4), and the spot diameter is around 25 μm. The large laser spot ensures that the whole GaN nanowires are efficiently pumped. A quarter-wave plate is used to change the linear polarized laser source to be circularly polarized. The emission from the plasmonic devices is collected by the same objective with the back-scattering configuration and analysed by the spectrometer. A polarization analyser is placed before spectrometer entrance to select the emission polarization. For low-temperature lasing spectroscopy, a liquid N 2 continuous-flow microscopy cryostat was used and the samples were pasted to the cold finger of the cryostat with silver paste to ensure good thermal conduction. The time-resolve photoluminescence (TRPL) spectra of an individual plasmonic device were investigated using a home-built confocal microscope system. Both the excitation pulses and emission light was coupled and collected through a × 20 microscope objective (numerical aperture=0.45). The pump pulses (650 nm) were generated from an optical parametric amplifier (Light Conversion TOPAS) that was pumped by a 1-kHz regenerative amplifier (Coherent Legend; centre wavelength: 800 nm; pulse width: 150 fs; power: 1 mJ per pulse), which was in turn seeded by an 80-MHz Coherent Vitesse oscillator. The emission signal was collected by an Optronis Optoscope streak camera system (for TRPL measurement). The streak camera system has an ultimate temporal resolution of ~10 ps when operated at the shortest time window of 330 ps. Numerical calculations on modal eigenvalues, loss and area The cross-section waveguide-mode properties (effective indices and field distributions) of the GaN–SiO 2 –Al configuration and the configurations of GaN nanowire sitting on SiO 2 substrate were calculated using finite-element method (COMSOL). The refractive indices of GaN and SiO 2 are 2.65 and 1.46 at λ =370 nm, respectively. The eigenvalue solver was used to find modes. Full three-dimensional simulations using the above hybrid plasmonic mode or photonic mode as the input were performed to calculate the near-field electric field distribution and the far-field emission. Perfectly matched layers were used to mimic the open-boundary conditions. In photonic mode simulation, the thickness of SiO 2 film is assumed to be infinite. After we obtained the eigenvalues of the hybrid waveguide mode, the modal loss can be evaluated using the propagation length defined as the length a mode travels before decaying to e −1 of its original power, such that Λ=1/2 Im{ β }. The modal area is defined as the ratio of the total mode energy and its peak energy density, where is the energy density per unit length along the direction of propagation. | E ( r )| 2 and | H ( r )| 2 are the modal electric and magnetic field distributions, respectively; ε ( r ) is the material electric permittivity, μ 0 is the vacuum magnetic permeability. For dielectric materials (SiO 2 ), the material electric permittivity dispersion is disregarded, that is, d ( ε ( r ) ω )/d ω ≈ ε ( r ); whereas, d ( ε ( r ) ω )/d ω = ε ( r )+ ωdε ( r )/d ω for Al. Particularly, to compensate big metal loss in the plasmonic device, high carrier density and gain threshold will pull up the dispersion of the semiconductor (refs [9] , [10] 9, 10), therefore for GaN electric permittivity dispersion is considered, that is, d ( ε ( r ) ω )/d ω = ε ( r )+ ωdε ( r )/d ω . Numerical calculations on local Purcell factor To study the local enhancement of the exciton recombination rate due to a broadband Purcell effect, we calculated the local Purcell factor following the procedure reported previously [9] . The emission rate for a dipole emitter at position r within the GaN nanowire is split into components corresponding to the enhancement of the emission rate of radiation modes, F R , SPP modes, F SPP and the lossy surface waves (LSW), F LSW . Assuming that only a small modification of the radiative emission rate occurs, we have F R ≈1. The SPP contribution to the Purcell factor is averaged over both of the available dipole orientations, , where F SPP, μ ( r )=3 n g ( λ /2 n 0 ) 2 / πn s A SPP, μ ( r ) is the SPP enhanced emission rate Purcell factor with an orientation along the μ direction, n g is the SPP group velocity, n s is the refractive index of semiconductor GaN, and is a measure of the mode area for a given dipole orientation and position. Lossy surface waves are associated with high in-plane momentum leaky waves of the metal and are extremely localized, , where , ε m and ε s are the permittivity of metal Al and semiconductor GaN, respectively, h is the insulator SiO 2 gap height. Confinement factor and lasing threshold To achieve lasing, the threshold condition requires the modal gain per unit length should be greater than the modal loss per unit length and the average reflection loss per unit length. The bulk GaN gain threshold should be . Γ s =2 n g W e s / n s W, (refs 47 , 48 ) where are the confinement factors of the semiconductor GaN nanowire and the metal region, respectively, is the bulk material gain coefficient of semiconductor GaN, is the bulk material absorption coefficient of metal with n m being its real part of the refractive index, L is the length of the nanowire and R is the modal reflection efficiency by the end facet. The gain and absorption coefficients are in unit of inverse length. As a result, Since has been obtained from the data of Johnson and Christy [28] (ref. 28), L has been readily measured, and R has been calculated using three-dimensional finite-element method simulation, the key to calculate the lasing threshold lies in the confinement factor. For the structure with GaN nanowire-edge length of 100 nm, at λ =370 nm, , Λ =0.58 μm, Γ s =3.4240, Γ m =0.011, R =0.15, . The measured nanowire length L =15 μm, and accordingly −2/ L ln R =2.529 × 10 3 cm −1 . Then we obtained the bulk GaN gain threshold, , which is smaller than the expected gain of GaN nanowire from literature. How to cite this article : Zhang, Q. et al. A room temperature low-threshold ultraviolet plasmonic nanolaser. Nat. Commun. 5:4953 doi: 10.1038/ncomms5953 (2014).